Signalling properties of inorganic polyphosphate in the mammalian brain Inorganic polyphosphate is known to be present in the mammalian brain at micromolar concentrations. Here we show that polyphosphate may act as a gliotransmitter, mediating communication between astrocytes. It is released by astrocytes in a calcium-dependent manner and signals to neighbouring astrocytes through P2Y 1 purinergic receptors, activation of phospholipase C and release of calcium from the intracellular stores. In primary neuroglial cultures, application of polyP triggers release of endogenous polyphosphate from astrocytes while neurons take it up. In vivo , central actions of polyphosphate at the level of the brainstem include profound increases in key homeostatic physiological activities, such as breathing, central sympathetic outflow and the arterial blood pressure. Together, these results suggest a role for polyphosphate as a mediator of astroglial signal transmission in the mammalian brain. Brain function relies on fast and effective communication between cells, and molecules of diverse origin and chemical structure (amino acids, monoamines, gases, purines and others) have been shown to mediate signal transmission within and between interconnected neuronal and glial networks. Inorganic polyphosphates (polyPs) are linear polymers of orthophosphate residues linked by phosphoanhydride bonds that have been identified in a variety of mammalian tissues, including the central nervous system (CNS; 25–120 μM) [1] , [2] . For many years, polyP was thought to be a ‘fossil’ molecule with no clear function in higher organisms, as no specific mammalian enzymes responsible for synthesis and degradation of polyP were identified. Recently, we showed that polyP can be produced by mammalian mitochondria [3] and has an important role in the mechanisms underlying Ca 2+ -dependent cell death [4] . PolyP was also identified as one of the key modulators of platelet-mediated pro-inflammatory and pro-coagulant disorders [5] . Furthermore, polyP has been shown to modulate the activities of TRPA1 and TRPM8 channels [6] , [7] , suggesting that it may be involved in neuronal signalling. Here we demonstrate previously unappreciated signalling properties of polyP in the mammalian CNS. The data obtained suggest that polyP acts as a gliotransmitter through astroglial purinergic receptors, more specifically P2Y 1 , leading to activation of phospholipase C (PLC) and release of Ca 2+ from the internal stores. Application of polyP to primary neuroglial cultures initiates further release of polyP from astrocytes while neurons take it up. This is dependent on Ca 2+ , as the Ca 2+ ionophore ionomycin also releases polyP. In vivo , central actions of polyP are consistent with astroglial activation, and at the level of the brainstem include profound increases in breathing, central sympathetic outflow and the arterial blood pressure. PolyP induces a calcium signal in cultured astrocytes As activation of brain cells is marked by increases in intracellular Ca 2+ ([Ca 2+ ] c ), we determined whether application of polyP, at concentrations which have been found in the mammalian brain (0.1–100 μM) [1] , has an effect on [Ca 2+ ] c in cultured neurons and astrocytes. In the rat neuroglial cultures, the majority of astrocytes and a small fraction of neurons responded with increases in [Ca 2+ ] c , following application of short (S; Supplementary Fig. S1a ), medium (M; Fig. 1a ) or long (L; Supplementary Fig. S1b ) polyP (14, 60, 130 phosphates, respectively). There were no significant differences in the amplitudes of Ca 2+ signals evoked in astrocytes by polyP of different lengths. However, the number of astrocytes that responded to polyP varied from 19 to 74%, depending on the concentration and length of polyP applied ( Supplementary Fig. S1c–e ), whereas only a small fraction (3%, n =120) of neurons responded even to high concentrations (50 μM) of polyP ( Fig. 1b ). These polyP-evoked responses were observed in the midbrain, hippocampal, as well as cortical cultures. For consistency, all subsequent experiments were performed using M-polyP at a concentration of 50 μM, whereas the results have been independently confirmed using L-polyP. Further characterization of polyP-induced signalling indicated that the recovery time of the evoked Ca 2+ transients is in the range of 700–1,000 s, as assessed by repeated applications of polyP to the same preparation ( Supplementary Fig. S1f–h ). Consistent with these results, we found that the responses originate from Ca 2+ recruitment from the internal stores, as removal of extracellular Ca 2+ (Ca 2+ -free media containing 0.5 mM EGTA; n =279; Fig. 1c ) did not block polyP-evoked responses in astrocytes. This was confirmed by complete inhibition of polyP-induced Ca 2+ signal after emptying reticulum Ca 2+ stores (1 μM thapsigargin-induced SERCA inhibition; n =101; Fig. 1d ). The PLC inhibitor U73122 (5 μM) also completely blocked polyP-induced Ca 2+ responses in astrocytes ( Fig. 1e ; n =739), suggesting that PLC is recruited, leading to IP 3 generation and mobilization of internal Ca 2+ stores. Upstream of PLC activation, we were able to identify the receptor mediating the observed actions of polyP. Blockade of purinergic receptors using the broad spectrum P2 receptor antagonist suramin (500 μM; n =245; Fig. 1f ) was found to completely abolish polyP-evoked [Ca 2+ ] c responses in cultured astrocytes. 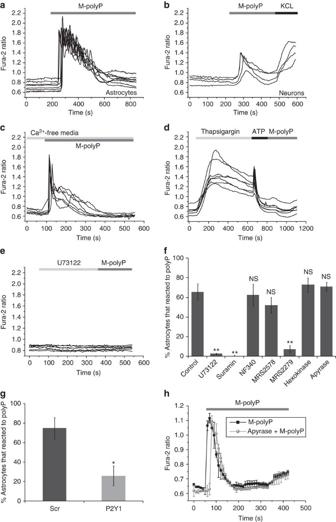Figure 1: PolyP induces Ca2+responses in neurons and astrocytes. Medium polyP (50 μM) induces [Ca2+]cchanges in hippocampal astrocytes (a) and neurons (b) as seen by an increase in the ratio of the Ca2+dye Fura-2. KCl (50 mM) was added at the end of the experiment for cellular (neuronal) identification. (c) Removal of external Ca2+(Ca2+-free medium with 0.5 mM EDTA) does not abolish polyP-induced Ca2+responses in astrocytes in response to 50 μM M-polyP. (d) Depletion of intracellular Ca2+stores with thapsigargin (1 μM) and ATP (100 μM) abolishes M-polyP (50 μM)-induced Ca2+responses in astrocytes. (e) M-polyP (50 μM)-induced [Ca2+]cresponses are inhibited in the presence of the PLC inhibitor U73122 (5 μM). Shown are representative traces from at least three independent experiments. (f) PLC inhibitor U73122, P2 receptor antagonist suramin (500 μM), and specific P2Y1receptor antagonist MRS2279 (50 μM) blocked the polyP-induced [Ca2+]cresponses, whereas the ATP-degrading enzymes hexokinase and apyrase (each 25 U ml−1) and the specific P2Y6, P2Y11receptor inhibitors (MRS2578 (10 μM) and NF340 (10 μM), respectively) had no effect. All experiments were performed using 50 μM M-polyP. Error bars represent s.e.m.,n>100 cells for each condition, **P<0.005, N.S., not significant. (g) Knockdown of the P2Y1receptor using shRNA suppressed the polyP-induced Ca2+signal (compared with a scrambled control, Scr). Error bars represent s.e.m.,n=201 for P2Y1andn=51 for Scr, *P<0.05. (h) Pre-incubation of cells with apyrase (25 U ml−1) did not affect the amplitude of M-polyP (50 μM)-induced Ca2+signal. Student’st-test was used to asses statistical significance. Figure 1: PolyP induces Ca 2+ responses in neurons and astrocytes. Medium polyP (50 μM) induces [Ca 2+ ] c changes in hippocampal astrocytes ( a ) and neurons ( b ) as seen by an increase in the ratio of the Ca 2+ dye Fura-2. KCl (50 mM) was added at the end of the experiment for cellular (neuronal) identification. ( c ) Removal of external Ca 2+ (Ca 2+ -free medium with 0.5 mM EDTA) does not abolish polyP-induced Ca 2+ responses in astrocytes in response to 50 μM M-polyP. ( d ) Depletion of intracellular Ca 2+ stores with thapsigargin (1 μM) and ATP (100 μM) abolishes M-polyP (50 μM)-induced Ca 2+ responses in astrocytes. ( e ) M-polyP (50 μM)-induced [Ca 2+ ] c responses are inhibited in the presence of the PLC inhibitor U73122 (5 μM). Shown are representative traces from at least three independent experiments. ( f ) PLC inhibitor U73122, P2 receptor antagonist suramin (500 μM), and specific P2Y 1 receptor antagonist MRS2279 (50 μM) blocked the polyP-induced [Ca 2+ ] c responses, whereas the ATP-degrading enzymes hexokinase and apyrase (each 25 U ml −1 ) and the specific P2Y 6 , P2Y 11 receptor inhibitors (MRS2578 (10 μM) and NF340 (10 μM), respectively) had no effect. All experiments were performed using 50 μM M-polyP. Error bars represent s.e.m., n >100 cells for each condition, ** P <0.005, N.S., not significant. ( g ) Knockdown of the P2Y 1 receptor using shRNA suppressed the polyP-induced Ca 2+ signal (compared with a scrambled control, Scr). Error bars represent s.e.m., n =201 for P2Y 1 and n =51 for Scr, * P <0.05. ( h ) Pre-incubation of cells with apyrase (25 U ml −1 ) did not affect the amplitude of M-polyP (50 μM)-induced Ca 2+ signal. Student’s t -test was used to asses statistical significance. Full size image PolyP-induced calcium signalling by P2Y 1 receptor activation To identify the specific P2 receptor through which polyP exerts its action, we tested several more selective P2 receptor antagonists. As polyP-evoked increases in intracellular [Ca 2+ ] c originate from the endoplasmic reticulum, the ionotropic (P2X) purinoreceptors could be ruled out. Selective antagonists of P2Y 1 , P2Y 6 , P2Y 11 (MRS2279 (ref. 8 ) (500 nM–50 μM), MRS2578 (refs 9 , 10 ) (10 μM) and NF340 (ref. 10 ) (10 μM), respectively) were applied before testing the effects of polyP. MRS2578 and NF340 were ineffective ( n =109 and n =295, respectively ( Fig. 1f )); however, blockade of polyP-induced Ca 2+ responses with MRS2279 suggested that activation of P2Y 1 receptors mediates polyP-induced effects. The number of cells that responded to application of polyP was greatly suppressed in cultures pre-treated with MRS2279 (50 μM n =803; Fig. 1f , 5 μM ( n =472) and 500 nM ( n =172); Supplementary Fig. S2a ). Knockdown of the P2Y 1 receptor using specific short hairpin RNA (shRNA) led to a reduced expression of the targeted protein ( Supplementary Fig. S2b,c ) as compared with a non-targeting shRNA (Scr). The loss of P2Y 1 receptor expression resulted in a significant reduction in the number of cells that responded to application of polyP (P2Y 1 , n =201; Scr, n =51; Fig. 1g ). PolyP-evoked responses do not appear to be mediated by prior release of ATP, as pre-treatment of cultures with ATP-degrading enzymes hexokinase (25 U ml −1 ) or apyrase (25 U ml −1 ; n =96 and n =101, respectively; Fig. 1f ) had no effect on the numbers of responding cells and amplitudes of the evoked Ca 2+ transients ( Fig. 1h ). Furthermore, ATP (100 μM), but not polyP-evoked Ca 2+ responses, were effectively blocked by apyrase ( Supplementary Fig. S2d ), confirming the efficacy of this approach in blocking ATP actions. Collectively, these data suggest that polyP may act on purinergic P2Y 1 receptors, leading to activation of PLC and recruitment of Ca 2+ from the internal stores. PolyP evokes release of endogenous polyP PolyP can be visualized in living cells after binding to the fluorescent dye (4′,6-diamidino-2-phenylindole) DAPI (polyP-DAPI) [5] , [11] . Astrocytes loaded with DAPI show an uneven polyP distribution in different cellular compartments—the nucleus, lysosomes, mitochondria and cytoplasmic vesicle-like structures ( Fig. 2a ; Supplementary Fig. S3a ; see also [3] , [4] , [11] , [12] ). Application of polyP to DAPI-loaded neuroglial cultures resulted in an immediate loss of vesicular polyP-DAPI staining in astrocytes and a concomitant increase in extracellular polyP (astrocytes n =22; Fig. 2a–c ), indicating release of polyP. This was accompanied by an increase in polyP-DAPI fluorescence in neurons (increase in fluorescence by 63.6±4.3% in neurons, n =32 compared with a decrease in astrocytes by 46.4±3.9%, n =39), suggesting that polyP is taken up by neurons ( Fig. 2d ). As the plasma membrane is impermeable to polyP, these observations suggest that polyP is cleared from the extracellular space by neuronal uptake (via an unknown transporter mechanism) and indicate polyP-evoked polyP release. Interestingly, polyP release was also evoked when the Ca 2+ ionophore ionomycin was applied ( n =29; Fig. 2f–i ), suggesting that the mechanism of polyP release is Ca 2+ -dependent. PolyP- and ionomycin-evoked polyP releases were confirmed with TBE-Urea gel electrophoresis and staining with DAPI ( Supplementary Fig. S3b ). 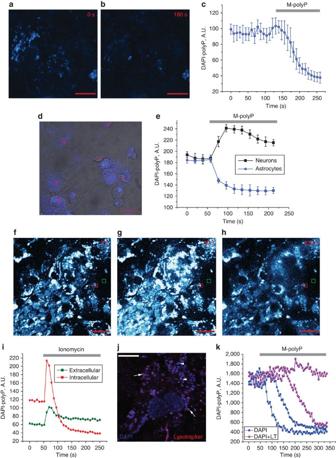Figure 2: Uptake and release of polyP in primary neuroglial co-cultures. PolyP can be detected in vesicle-like structures in astrocytes using DAPI (DAPI-polyP) (a). Application of M-polyP (50 μM) to DAPI-loaded neuroglial cultures induces release of polyP as seen by a decrease in intracellular vesicular DAPI-polyP (a–c). Error bars represent s.e.m.n=93 cells. Shown are representative images from two time points and the mean trace. Scale bar, 10 μm. PolyP released from astrocytes (a) upon stimulation with M-polyP (50 μM) is taken up by neurons (n) as seen by DAPI-polyP (d). (d) Bright-field image combined with DAPI-polyP staining (blue). Scale bar, 20 μm. (e) Representative mean traces from neurons and astrocytes. Error bars represent s.e.m.n=54 neurons andn=61 astrocytes. (f–i) Application of ionomycin (5 μM) induces release of vesicular polyP from cortical astrocytes. Shown are representative images from three time points (0, 60, 250 s) (f–h) and the corresponding traces (i). (j) Loading of neuroglial cultures with DAPI and Lysotracker (LT) simultaneously indicates partial colocalization of DAPI-polyP with lysosomes (arrows), whereas other DAPI-polyP vesicles do not stain with LT (arrow heads). Scale bar, 10 μm. (k) PolyP is released from a proportion of LT and DAPI co-stained vesicles upon addition of 50 μM M-polyP. Figure 2: Uptake and release of polyP in primary neuroglial co-cultures. PolyP can be detected in vesicle-like structures in astrocytes using DAPI (DAPI-polyP) ( a ). Application of M-polyP (50 μM) to DAPI-loaded neuroglial cultures induces release of polyP as seen by a decrease in intracellular vesicular DAPI-polyP ( a – c ). Error bars represent s.e.m. n =93 cells. Shown are representative images from two time points and the mean trace. Scale bar, 10 μm. PolyP released from astrocytes (a) upon stimulation with M-polyP (50 μM) is taken up by neurons (n) as seen by DAPI-polyP ( d ). ( d ) Bright-field image combined with DAPI-polyP staining (blue). Scale bar, 20 μm. ( e ) Representative mean traces from neurons and astrocytes. Error bars represent s.e.m. n =54 neurons and n =61 astrocytes. ( f – i ) Application of ionomycin (5 μM) induces release of vesicular polyP from cortical astrocytes. Shown are representative images from three time points (0, 60, 250 s) ( f – h ) and the corresponding traces ( i ). ( j ) Loading of neuroglial cultures with DAPI and Lysotracker (LT) simultaneously indicates partial colocalization of DAPI-polyP with lysosomes (arrows), whereas other DAPI-polyP vesicles do not stain with LT (arrow heads). Scale bar, 10 μm. ( k ) PolyP is released from a proportion of LT and DAPI co-stained vesicles upon addition of 50 μM M-polyP. Full size image Interestingly, polyP has been found in lysosomes [12] . We found partial colocalization of polyP-DAPI with the lysosomal marker LysoTracker ( Fig. 2j ), which selectively labels lysosomes in cultured astrocytes [13] . Stimulation of cells with exogenous polyP induces release of DAPI-polyP from some but not all lysosomes, although predominantly polyP is released from non-lysosomal vesicle-like compartments ( Fig. 2k ). These data indicate that astrocytes can release polyP via Ca 2+ -dependent exocytotic mechanism. Ca 2+ -dependent release of endogenous polyP As an increase in [Ca 2+ ] c induces release of polyP, we next determined whether Ca 2+ excitation of astrocytes results in a release of endogenous polyP and polyP-mediated activation of neighbouring cells. We used caged Ca 2+ (np-EGTA) and flash photolysis to evoke an increase in intracellular Ca 2+ in an individual cell (flashed). Ca 2+ uncaging in a single astrocyte triggered an increase in intracellular [Ca 2+ ] c in neighbouring (non-flashed) astrocytes ( Fig. 3c ), even in the presence of apyrase (25 U ml −1 ; Fig. 3a ) and inhibitors of either ionotropic or metabotropic glutamate receptors, including CNQX (20 μM; n =5 experiments), MK-801 (10 μM; n =9 experiments) or (S)-MCPG (50 μM; n =6 experiments). However, suramin (500 μM) or MRS2279 (5 and 50 μM; Fig. 3d and Supplementary Fig. S2e ) blocked Ca 2+ responses in neighbouring cells, suggesting that Ca 2+ -dependent release of polyP from astrocytes induces a Ca 2+ signal in neighbouring cells through activation of P2Y 1 receptors. 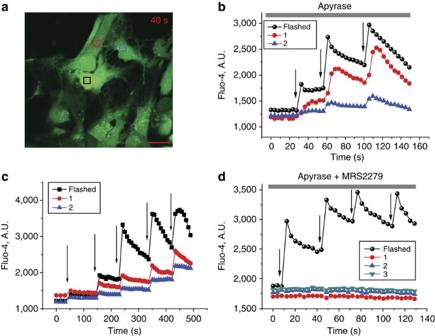Figure 3: Ca2+-induced polyP release. Uncaging of Ca2+by ultraviolet flash (depicted by black arrows and a black square and trace) in a single cultured astrocyte induces Ca2+signal in neighbouring cells in the presence of apyrase (25 U ml−1; red and blue squares and traces) (a,b). Scale bar, 20 μm. (c) Removal of apyrase from the medium had no effect on the amplitude of the induced Ca2+signal (black arrows indicate time of the flash). (d) The transmission of the signal can be blocked by inhibition of the P2Y1receptors with MRS2279 (50 μM). Figure 3: Ca 2+ -induced polyP release. Uncaging of Ca 2+ by ultraviolet flash (depicted by black arrows and a black square and trace) in a single cultured astrocyte induces Ca 2+ signal in neighbouring cells in the presence of apyrase (25 U ml −1 ; red and blue squares and traces) ( a , b ). Scale bar, 20 μm. ( c ) Removal of apyrase from the medium had no effect on the amplitude of the induced Ca 2+ signal (black arrows indicate time of the flash). ( d ) The transmission of the signal can be blocked by inhibition of the P2Y 1 receptors with MRS2279 (50 μM). Full size image PolyP evokes profound cardiorespiratory responses in vivo Finally, we established the effects of polyP in vivo . Using anaesthetized and artificially ventilated rats, we found that application of polyP to the chemosensory areas located on the ventral surface of the brainstem evokes profound increases in key cardiorespiratory variables—breathing (by 241±37%; P =0.030; n =6), central sympathetic outflow (by 101±20%; P =0.011; n =6), heart rate (by 69±10 beats min −1 ; P =0.003; n =6) and the arterial blood pressure (by 41±5 mm Hg; P =0.002; n =6; Fig. 4a ). These effects of polyP lasted for 31±4 min ( n =6). MRS2279 (50 μM) or broad spectrum P2 receptor antagonist PPADS (pyridoxal-phosphate-6-azophenyl-2',4'-disulphonate; 100 μM) applied on the ventral surface of the brainstem 5 min before polyP had no effect on resting level of cardiorespiratory activity ( Supplementary Fig. S4 ), but dramatically reduced the magnitude of polyP-evoked responses ( Fig. 4b ). This is consistent with the effects of polyP on the brainstem subpial astrocytes and glia limitants capable of driving these changes in response to physiological stimulation (such as decreased pH) [14] . These data indicate that the effects of exogenously applied polyP on respiratory and cardiovascular activities are remarkably similar to that of another notable gliotransmitter—ATP [15] . 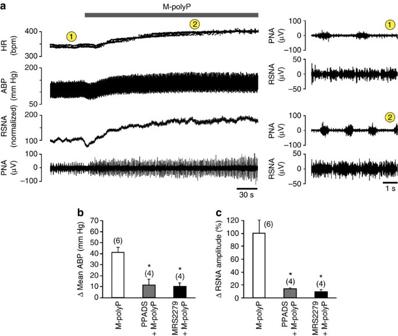Figure 4: Effects of polyPin vivo. Application of M-polyP (50 μM) to the ventral surface of the brainstem increases heart rate (HR), arterial blood pressure (ABP), renal sympathetic nerve activity (RSNA) and phrenic nerve activity (PNA) (a). Expanded traces of PNA and RSNA on the right depict the activities before and after application of polyP. Time points are indicated by numbers (1) and (2) on the time-condensed trace on the left. The effects of M-polyP on the ABP (b) and RSNA (c)in vivoare blocked by pre-treatment with P2 receptor antagonists PPADS (100 μM) or MRS2279 (50 μM). Values are means±s.e.m. Numbers in parentheses indicate sample sizes. *P<0.01 compared with the effect of M-polyP applied alone (ANOVA followed by Tukey–Kramer’spost hoctest). Figure 4: Effects of polyP in vivo . Application of M-polyP (50 μM) to the ventral surface of the brainstem increases heart rate (HR), arterial blood pressure (ABP), renal sympathetic nerve activity (RSNA) and phrenic nerve activity (PNA) ( a ). Expanded traces of PNA and RSNA on the right depict the activities before and after application of polyP. Time points are indicated by numbers (1) and (2) on the time-condensed trace on the left. The effects of M-polyP on the ABP ( b ) and RSNA ( c ) in vivo are blocked by pre-treatment with P2 receptor antagonists PPADS (100 μM) or MRS2279 (50 μM). Values are means±s.e.m. Numbers in parentheses indicate sample sizes. * P <0.01 compared with the effect of M-polyP applied alone (ANOVA followed by Tukey–Kramer’s post hoc test). Full size image In summary, our data show that polyP triggers strong activation (increases in intracellular Ca 2+ ) of the majority of astrocytes, irrespective of the brain region examined and of a small proportion of CNS neurons. This is consistent with the data showing that polyP signals via activation of P2Y receptors, more specifically P2Y 1 , which are found to be expressed predominantly by astroglia [16] . Interestingly, P2Y 1 receptors are known to be activated by a diverse array of molecules, including ADP and ATP, as well as by diadenosine polyP, a molecule containing two adenosines and up to seven phosphate groups [17] . Furthermore, specific residues of the P2Y 1 receptor complex are known to interact with phosphate groups [18] . P2Y 1 receptors are not only expressed in the CNS but also in many other tissues, including smooth muscle, bone and platelets [16] . Interestingly, polyP has been shown to be released by activated platelets [5] . Whether polyP-induced polyP release triggered via activation of P2Y 1 receptors is a common mechanism remains to be determined. In neuroglial cultures, activation of astrocytes leads to the release of polyP, which is cleared from the extracellular space by neuronal uptake. Whether this is only lysosomal release, as our data suggest, or also occurs via vesicular mechanisms which similarly has been implicated in the release of gliotransmitters (such as ATP) from astrocytes [19] , remains to be seen. It is also possible that other transmitters such as ATP and diadenosine polyP are being released simultaneously with polyP. Furthermore, there are probably other P2Y receptors to which polyP can bind, as loss of P2Y 1 activity does not fully block polyP-induced Ca 2+ signalling. The actions of polyP on the brainstem respiratory and autonomic circuits stimulate breathing, increase sympathetic outflow and raise arterial blood pressure (in a P2Y 1 receptor-dependent manner), demonstrating potential functional significance of polyP-mediated signalling in vivo . Interestingly, although the polyP-mediated effects are similar to those of ATP [14] they are not dependent on ATP, suggesting that ATP and polyP may have common downstream targets. These data suggest that activated astrocytes in the mammalian CNS are capable of utilizing polyP as a gliotransmitter, which may have an important role in the control of vital behaviours in which astroglia are implicated. Cell culture Mixed cultures of hippocampal, cortical or midbrain neurons and glial cells were prepared as described previously [20] , with modifications, from Sprague-Dawley rat pups 3 days postpartum (UCL breeding colony). Hippocampi, cortex and midbrain were removed into ice-cold HEPES buffered salt solution (Ca 2+ , Mg 2+ -free; Gibco-Invitrogen, Paisley, UK). The tissue was minced and trypsinized (0.25% for 15 min at 37 °C), triturated and plated on poly- D -lysine-coated coverslips and cultured in neurobasal A medium (Gibco-Invitrogen) supplemented with B-27 (Gibco-Invitrogen) and 2 mM L -glutamine. Cultures were maintained at 37 °C in a humidified atmosphere of 5% CO 2 and 95% air, fed once a week and maintained for a minimum of 12 days before experimental use, to ensure the expression of glutamate and other receptors. Neurons were easily distinguishable from glia: they appeared phase bright, had smooth rounded somata and distinct processes, and lay just above the focal plane of the glial layer. Cells were used at 14–21days in vitro . A lentiviral pGIPZ shRNA vector encoding shRNA targeting P2Y 1 receptor and a negative, non-targeting shRNA control (scr) vector, both of which also encode green fluorescent protein as a reporter protein, were obtained from a commercial provider (Thermo Fisher). With HEK 293T cells, the pGIPZ and negative shRNA vectors were packaged into a lentivirus using a three plasmid transfection procedure [21] . Primary neuroglial cultures were then transduced with the packaged pGIPZ shRNA lentivirus. In brief, cells on one 6-cm dish were incubated in 2 ml DMEM containing the virus for 4 h. After 4 h, the medium was exchanged for normal neurobasal A medium, and the cultures were incubated for an additional 72 h. Transduction efficiency was estimated to be between 30–80% by direct visualization of green fluorescent protein expression. Imaging [Ca 2+ ] c and polyP Primary neurons and astrocytes were loaded for 30 min at room temperature with 5 μM fluo-4, 5 μM fura-2 AM, 5 μM lysotracker Red DND-99 or 0.5 μM DAPI (Molecular Probes, Eugene, OR), and 0.005% Pluronic in a HEPES buffered salt solution composed (in mM) 156 NaCl, 3 KCl, 2 MgSO 4 , 1.25 KH 2 PO 4 , 2 CaCl 2 , 10 glucose and 10 HEPES, pH adjusted to 7.35 with NaOH. Ca 2+ -free medium contained 0.5 mM EGTA and no Ca 2+ . PolyP standards (sodium salt with polyP content of 60%) were provided by Dr T Shiba (Regenetiss, Inc., Japan). Fluorescent Ca 2+ measurements using fura-2 were obtained on an epifluorescence inverted microscope equipped with a X20 fluorite objective. Changes in [Ca 2+ ] c were monitored in single cells using excitation light provided by a Xenon arc lamp, the beam passing monochromator at 340, 380 nm (Cairn Research, Kent, UK). Emitted fluorescence light was reflected through a 515-nm long pass filter to a cooled CCD camera (Retiga, QImaging, Canada) and digitized to 12 bit resolution. All imaging data were collected and analysed using software from Andor (Belfast, UK). The fura-2 data have not been calibrated in terms of [Ca 2+ ] c because of the uncertainty arising from the use of different calibration techniques. When inhibitors were used, control recordings were first performed in the absence of the antagonist. Confocal images in combination with flash photolysis were obtained using a Zeiss 510 UV–vis CLSM equipped with a META detection system and a X40 oil immersion objective. For flash photolysis experiments, caged Ca 2+ , 10 μM o -nitrophenyl EGTA, AM (NP-EGTA, AM) was loaded at the same time as fluo-4 (ref. 22 ). Each ultraviolet flash was targeting a single cell. The 488-nm Argon laser line was used to excite fluo-4, which was measured at 505–550 nm. Illumination intensity was kept to a minimum (at 0.1–0.2% of laser output) to avoid phototoxicity and the pinhole set to give an optical slice of ~2 μm. Confocal images of DAPI-polyP and Lysotracker staining were obtained using a Zeiss 710 LSM equipped with a META detection system and a X40 oil immersion objective. DAPI emission spectra were measured using 405 nm laser for excitation. The specific DAPI-polyP emission signal was measured above 550 nm, using the Zeiss ‘META’ system and presented as arbitrary units (A.U.) [4] , [11] . A separation of the DAPI–DNA and DAPI-polyP signal is shown in Supplementary Figure S2a . Lysotracker red was excited at 561 nm and measured at up to 580 nm. The representative images show the typical regions chosen for the analysis in each case. Several regions from neurons and astrocytes, as well as from the extracellular media, were analysed and the intensity averaged for each type of region. All data presented were obtained from at least five coverslips and two different cell preparations. The numbers of cells analysed in each experiment are indicated in the text. In vivo experiments Experiments were performed on 12 male Sprague-Dawley rats (300–340 g) and carried out in accordance with the UK Animals (Scientific Procedures) Act, 1986. The rats were anaesthetized with urethane (1.6 g kg −1 , intraperitoneally). Adequate anaesthesia was ensured by maintaining stable levels of arterial blood pressure, heart and central respiratory rate. The femoral artery and vein were cannulated for measurement of arterial blood pressure and administration of anaesthetic, respectively. The trachea was cannulated, the animal was vagotomized and ventilated with a mixture of 50% oxygen and 50% nitrogen using a positive pressure ventilator (Harvard rodent ventilator, model 683) with a tidal volume of ~2 ml and a ventilator frequency similar to spontaneous frequency (~60 strokes per min). The animal was then injected with gallamine triethiodide (Flaxedil, 40 mg kg −1 , intravenously; then 10 mg kg −1 h −1 , intravenously) and was placed in a stereotaxic frame. The ventral surface of the brainstem was exposed as described previously [14] , [23] , [24] . Activities of the phrenic and renal nerves were recorded as indicators of central respiratory and sympathetic drives. Renal sympathetic nerve activity was integrated and smoothed with a time constant of 10 s (Spike 2 software, Cambridge Electronic Design Ltd, Cambridge, UK). The body temperature was maintained with a servo-controlled heating pad at 37.0±0.2 °C. PolyP (50 μM in saline) was applied to the exposed ventral surface of the brainstem and left on for the duration of the experiment. The effect of this treatment on the arterial blood pressure, heart rate, central respiratory and sympathetic drives was determined. PolyP-evoked changes in mean level of sympathetic activity were determined after normalization of renal sympathetic nerve activity with respect to both resting baseline level (100%) and complete absence of discharges (0%) following administration of a ganglionic blocker hexamethonium (20 mg; intravenously) at the end of the experiment. To determine whether P2 receptor activation mediates polyP effects on cardiorespiratory activity, MRS2279 (50 μM) or PPADS (100 μM) were applied to the ventral surface of the brainstem 5 min before polyP administration. Statistical analysis Statistical analysis was performed with the aid of Origin 8 (Microcal Software Inc., Northampton, MA, USA) software. Group data were compared using analysis of variance followed by the Tukey–Kramer’s post hoc test (for comparisons among three or more experimental groups) or Student’s t -test, as appropriate. Data are presented as means±s.e.m. Differences at P <0.05 were considered to be significant. How to cite this article: Holmström, K. M. et al . Signalling properties of inorganic polyphosphate in the mammalian brain. Nat. Commun. 4:1362 doi: 10.1038/ncomms2364 (2013).